Coexistence of the topological state and a two-dimensional electron gas on the surface of Bi2Se3 The surface of a topological insulator plays host to an odd number of linearly-dispersing Dirac fermions, protected against back-scattering by time-reversal symmetry. Such characteristics make these materials attractive not only for studying a range of fundamental phenomena in both condensed matter and particle physics, but also for applications ranging from spintronics to quantum computation. Here, we show that the single Dirac cone comprising the topological state of the prototypical topological insulator Bi 2 Se 3 can co-exist with a two-dimensional electron gas (2DEG), a cornerstone of conventional electronics. Creation of the 2DEG is tied to a surface band-bending effect, which should be general for narrow-gap topological insulators. This leads to the unique situation where a topological and a non-topological, easily tunable and potentially superconducting, metallic state are confined to the same region of space. Topological insulators are a recently discovered class of materials with fascinating properties: while the inside of the solid is insulating, fundamental symmetry considerations require the surfaces to be metallic [1] , [2] , [3] , [4] , [5] , [6] . The metallic surface states show an unconventional spin texture [7] , [8] , electron dynamics [9] , [10] , [11] , [12] and stability. Recently, surfaces with only a single Dirac cone dispersion have received particular attention [8] , [13] , [14] , [15] , [16] , [17] , [18] . These are predicted to play host to a number of novel physical phenomena such as Majorana fermions [19] , magnetic monopoles [20] and unconventional superconductivity [21] . Such effects will mostly occur when the topological surface state lies in close proximity to a magnetic or electric field, a (superconducting) metal, or if the material is in a confined geometry. The realisation of novel phenomena, but also the exploitation of the topological metallic states, will thus necessarily require the interfacing of topological insulators with other materials. In general, the introduction of such an interface will lead to an energy change (a bending) of the electronic bands in its vicinity, either caused by the presence of intrinsic surface/interface states or due to characteristic extrinsic defects, impurities or applied electric fields. It is essential to understand such effects not only for realising practical device applications, but also for correct interpretation of the results of surface-sensitive spectroscopic probes such as angle-resolved photoemission (ARPES) or scanning-tunnelling microscopy, which have become instrumental in the study of topological insulators. Here, we show that such a band bending near to the surface of the model topological insulator Bi 2 Se 3 gives rise to the formation of a two-dimensional electron gas (2DEG). The 2DEG, renowned from semiconductor surfaces and interfaces where it forms the basis of the integer and fractional quantum Hall effects [22] , [23] , two-dimensional superconductivity [24] , and a plethora of practical applications [25] , coexists with the topological surface state in Bi 2 Se 3 . This finding should be applicable to the other narrow-gap topological insulators, and will play an important role in both fundamental studies and realisation of device applications of these materials. 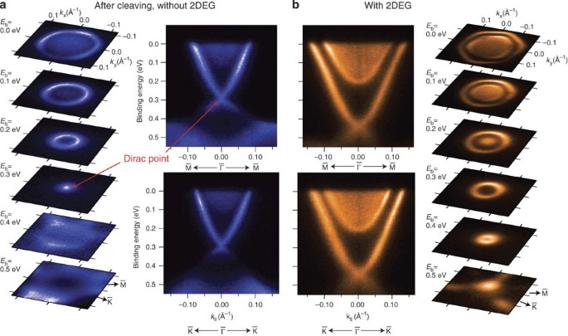Figure 1: Development of a surface 2DEG in Bi2Se3. (a) Electronic structure of Bi2Se3(0001), around 30 min after cleaving the sample, presented as cuts at different binding energies (Eb) (left) and dispersions along high-symmetry directions(right, top) and(right, bottom). The sharp V-like feature is the Dirac-like dispersion of the topological surface state. The valence band states are visible below the Dirac point and the diffuse intensity inside the Dirac cone is due to the filled bottom of the conduction band. (b) After three hours in vacuum, the chemical potential of the material is shifted, presumably due to the formation of defects. This shift is accompanied by the emergence of a sharp rim around the bottom of the conduction band. This is the spectral signature of the 2DEG near the surface. The constant energy contours of the topological state, the 2DEG, and the conduction band show a hexagonal shape near the Fermi energy. Inb, cuts at different binding energies are on the right, whereas dispersions along directionsare on the left, top andon the left, bottom, respectively. Angle-resolved photoemission The emergence of a 2DEG on the (0001) surface of Bi 2 Se 3 can be followed by ARPES, as shown in Figure 1 . Immediately after cleaving the sample, a sharp V-shaped topological state is observed in the gap. Features stemming from the bulk valence and conduction bands are also seen. The latter should not be observable by photoemission for an intrinsic semiconductor, but most as-grown Bi 2 Se 3 crystals turn out to be degenerately electron-doped [13] , [26] . Over a period of a few hours (depending on the sample temperature), spectral changes are observed. The chemical potential shifts gradually upwards, an effect which has been ascribed to a defect-induced downward band bending near the surface [13] . Eventually, we find that an intense and narrow rim emerges around the bottom of the conduction band ( Fig. 1b ). This state is assigned to a quantum-confined 2DEG, similar to what has been found for other narrow-gap semiconductors [27] , [28] . After about three hours the situation becomes more stable, with the sample gradually deteriorating but no further pronounced shifts of the chemical potential. We observed no change in low-energy electron diffraction (LEED) following creation of the 2DEG, with clear (1×1) LEED patterns observed both before and after its emergence (data not shown). This confirms that the downward band bending and consequent 2DEG formation is driven by the creation of extrinsic defects or the adsorption of impurities at the surface, rather than any surface reconstruction. Figure 1: Development of a surface 2DEG in Bi 2 Se 3 . ( a ) Electronic structure of Bi 2 Se 3 (0001), around 30 min after cleaving the sample, presented as cuts at different binding energies ( E b ) (left) and dispersions along high-symmetry directions (right, top) and (right, bottom). The sharp V-like feature is the Dirac-like dispersion of the topological surface state. The valence band states are visible below the Dirac point and the diffuse intensity inside the Dirac cone is due to the filled bottom of the conduction band. ( b ) After three hours in vacuum, the chemical potential of the material is shifted, presumably due to the formation of defects. This shift is accompanied by the emergence of a sharp rim around the bottom of the conduction band. This is the spectral signature of the 2DEG near the surface. The constant energy contours of the topological state, the 2DEG, and the conduction band show a hexagonal shape near the Fermi energy. In b , cuts at different binding energies are on the right, whereas dispersions along directions are on the left, top and on the left, bottom, respectively. Full size image Figure 1b also shows the dispersion of the topological state and the two-dimensional electron gas as constant energy cuts through a three-dimensional data set. The topological state has a circular constant energy contour near the Dirac point, but all the states (topological state, 2DEG and conduction band) show hexagonal contours near the Fermi level (435 meV above the Dirac point). This hexagonal warping of the topological state is apparent from its different Fermi wavevectors of k F =0.134(1) and 0.128(1) Å −1 along the directions, respectively. These observation are consistent with previous findings on Bi 2 Se 3 [29] , and on Bi 2 Te 3 [16] , [30] where the effect is more pronounced than here. For the conduction band and the 2DEG, the hexagonal shape implies a non-isotropic effective mass, a point we shall return to later. It is important to note the very different physical nature of the topological state and the 2DEG. The former is completely non-spin degenerate, apart from the Dirac point. As such, its quasiparticles are protected from back-scattering. The band structure does not permit the opening of energy gaps due to a small perturbation, or the formation of metal-insulator transitions in the form of charge-density waves, despite the strongly nested Fermi surface [31] (a spin-density wave would be permitted [30] ). The 2DEG, on the other hand, is almost certainly spin degenerate and could be prone to such instabilities. In fact, a hexagonal Fermi surface with its strong nesting has, to the best of our knowledge, not yet been observed for such a state. Most importantly, the existence of the 2DEG opens new decay channels for the topological state. An indication of this is the change in the linewidth of the latter. Immediately after cleaving the crystal, the topological state is found to be very narrow, of the order of Δ k ≈0.016(5) Å −1 at the Fermi level. If we interpret this width as a measure for the inverse mean free path on the surface l , this would correspond to l ≈70 Å [32] . This value is similar to what is found for highly-perfect epitaxial graphene [33] or cleaved high-temperature superconductors [34] . A long mean free path for the topological state is, of course, expected from the reduced phase space for scattering [35] . Once the 2DEG is established at the surface, the width of the topological state is increased to Δ k ≈0.019(5) Å −1 , while the 2DEG state is slightly wider (Δ k ≈0.024(5) Å −1 ). Apart from the presumably small increased number of defects near the surface, the increased width of the topological state is almost certainly related to the presence of the 2DEG itself, and the scattering processes now permitted between this and the topological state. The dimensionality of all of the observed states can be probed directly by performing ARPES measurements at different photon energies, thus varying the wave vector perpendicular to the surface, k z . 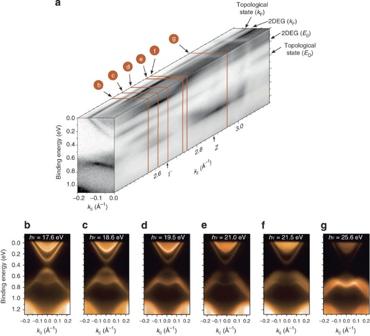Figure 2:kz-dependence of the electronic structure of Bi2Se3. (a) Three-dimensional representation of the electronic structure evolution of Bi2Se3withkz, determined from ARPES measurements taken at 181 photon energies between 14 and 32 eV, between 7 and 11 h after cleaving the sample. The bulk Γ and Z high symmetry points are indicated. Selected cuts (markedb–g) are shown, measured at photon energies of (b) 17.6, (c) 18.6, (d) 19.5, (e) 21.0, (f) 21.5, and (g) 25.6 eV. The measurements are taken at an angle enclosing 10.5° with thedirection. The complete data set is available asSupplementary Movie 1. Apart from intensity modulations due to matrix element effects, the topological state and the 2DEG do not change with photon energy (b–g), leading to marked linear features in (a) on thek||−kz(at the Fermi wavevectors,kF) and theEb−kzplanes (at the Dirac point, ED, and 2DEG band bottom,E0, respectively). This lack ofkzdispersion confirms their two-dimensional nature. A third linear feature in theEb−kzplane (Eb≈750 meV) is a surface state in the projected bulk band gap below the upper valence band (M-shaped feature, clearly visible in (g)). Figure 2a shows the result of such measurements, revealing the evolution of the electronic states on the Fermi surface, and within 1.1 eV of the Fermi level at , with k z . Selected measurements at different photon energies are also shown in Figure 2b–g (the full data set is available as Supplementary Movie 1 ). Both the topological state and the 2DEG do not disperse with k z , confirming their two-dimensional nature: they occur at the same energy and momentum in Figure 2b–g and give rise to linear features on both the k || − k z and the E b − k z planes ( Fig. 2a ). In contrast, a strong k z -dispersion of the bulk conduction (valence) band is evident, showing a maximum (minimum) in binding energy at the bulk Γ point at k z ≈2.65 Å −1 . This dispersion also explains the photon-energy-dependent 'filling' of the 2DEG contour, due to emission from bulk conduction band states ( Fig. 2b,d ). Figure 2: k z -dependence of the electronic structure of Bi 2 Se 3 . ( a ) Three-dimensional representation of the electronic structure evolution of Bi 2 Se 3 with k z , determined from ARPES measurements taken at 181 photon energies between 14 and 32 eV, between 7 and 11 h after cleaving the sample. The bulk Γ and Z high symmetry points are indicated. Selected cuts (marked b – g ) are shown, measured at photon energies of ( b ) 17.6, ( c ) 18.6, ( d ) 19.5, ( e ) 21.0, ( f ) 21.5, and ( g ) 25.6 eV. The measurements are taken at an angle enclosing 10.5° with the direction. The complete data set is available as Supplementary Movie 1 . Apart from intensity modulations due to matrix element effects, the topological state and the 2DEG do not change with photon energy ( b – g ), leading to marked linear features in ( a ) on the k || − k z (at the Fermi wavevectors, k F ) and the E b − k z planes (at the Dirac point, E D , and 2DEG band bottom, E 0 , respectively). This lack of k z dispersion confirms their two-dimensional nature. A third linear feature in the E b − k z plane ( E b ≈750 meV) is a surface state in the projected bulk band gap below the upper valence band (M-shaped feature, clearly visible in ( g )). Full size image While the topological and 2DEG states do not disperse in k z , these spectral features do show strong intensity variations with photon energy. Such a k z -dependence of the photoemission intensity of two-dimensional states is well known for metallic surface states, due to transition matrix element effects [36] , [37] . From Figure 2a , emission from the 2DEG is resonantly enhanced when the conduction band reaches its minimum at the bulk Γ point. In the E b − k z plane ( Fig. 2a ), another state is observed at a binding energy of ≈750 meV which does not disperse with k z . This corresponds to the M-shaped feature in the individual cuts, particularly pronounced in Figure 2g . We interpret this as another surface state, situated in a projected bulk band gap below the upper valence band near [14] . Similar to the 2DEG, emission from this state is resonantly enhanced when the bulk valence band dispersion reaches a minimum at the Z point ( k z ≈2.9 Å −1 ). 2DEG calculations The 2DEG on the surface is derived from the conduction band states, as indicated by its resonant enhancement near Γ, but confined in the z -direction due to a strong band bending near the surface. 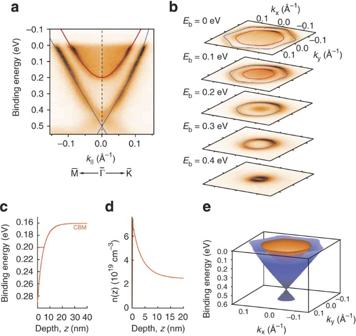Figure 3: Model calculations for the 2DEG and topological state. Coupled Poisson-Schrödinger calculations, incorporating conduction-band non-parabolicity and anisotropy of the effective mass, well reproduce the (a) dispersion and (b) constant energy contours of the 2DEG state. The downward bending of the conduction band at the surface and corresponding increase in near-surface carrier density (that is, the 2DEG formation) are shown in (c) and (d), respectively. The topological state is also reasonably characterized by model calculations describing hexagonal warping of the linear Dirac dispersion (a,b). Panel (e) shows the co-existence of the 2DEG (orange) and topological surface state (blue). We have performed model calculations to further substantiate the existence and origins of this 2DEG, as shown in Figure 3 . The near-surface band bending of the material and the dispersions of the resulting 2DEG states are calculated via a coupled solution of the Poisson and Schrödinger equations, based around the method described in ref. 38 . These calculations accurately reproduce the measured dispersion and constant energy contours of the 2DEG state, shown in Figure 3a,b , for a downward band bending at the surface of 0.13 eV ( Fig. 3c ), very similar to the shift of the Dirac point between the freshly cleaved sample and following the emergence of the 2DEG. It is this band bending which creates a potential well at the surface, causing quantum-confinement of the conduction band states, and development of the 2DEG. In the presence of a potential gradient, one may expect to observe a Rashba spin-splitting of the 2DEG state. However, from a simple model using the calculated band bending potential gradient, we estimate an upper limit for the Rashba splitting of only ∼ 0.004 Å −1 at the Fermi level, unlikely to be observable in practice. Figure 3: Model calculations for the 2DEG and topological state. Coupled Poisson-Schrödinger calculations, incorporating conduction-band non-parabolicity and anisotropy of the effective mass, well reproduce the ( a ) dispersion and ( b ) constant energy contours of the 2DEG state. The downward bending of the conduction band at the surface and corresponding increase in near-surface carrier density (that is, the 2DEG formation) are shown in ( c ) and ( d ), respectively. The topological state is also reasonably characterized by model calculations describing hexagonal warping of the linear Dirac dispersion ( a , b ). Panel ( e ) shows the co-existence of the 2DEG (orange) and topological surface state (blue). Full size image In addition to the main 2DEG state located ∼ 40 meV below the conduction band edge of the bulk (shown in Fig. 3c , and clearly apparent in the measured data ( Fig. 3a )), a second 2DEG state is predicted in the calculations at only ∼ 7 meV below the bulk band edge. This state is not shown in Figure 3 because, being so shallow, its wavefunction will be very extended in k z : consequently, we would expect this state to be very delocalized and to largely contribute to the diffuse intensity above the lower 2DEG state. However, we note that at some photon energies, a second state is discernible above the 2DEG band bottom (for example, Fig. 2e,f ). This second state is situated approximately 35 meV above the band bottom of the main 2DEG state, and so would be consistent with a second very shallow state as predicted by the calculations. The hexagonal Fermi surface contour of the 2DEG state implies an anisotropic in-plane effective mass, and we find values of 0.122 m 0 and 0.109 m 0 along , respectively. The 2DEG state also exhibits some deviations from parabolicity. We attribute this to a k · p interaction [39] between the conduction and valence bands, which we include within our calculations. A k · p model has also been proposed to describe the hexagonal warping of the topological surface state in Bi 2 Te 3 [30] . This model reproduces the dispersions and constant energy contours of the topological state observed here reasonably well ( Fig. 3a,b ), although the magnitude of the hexagonal warping term is approximately a factor of 2.3 smaller than that estimated from the measured Fermi velocity and wavevector, using the formalism within ref. 30 . The model calculations confirm the experimental findings presented above that a downward band bending at the surface of Bi 2 Se 3 induces a two-dimensional electron gas, that co-exists with the topological surface state ( Fig. 3e ). This suggests the possibility to modulate the 2DEG density via control of the band bending, either through absorption of elemental or molecular species on the clean surface, or via a gate electrode. Such a scheme could potentially be used to obtain a switchable metallic, and possibly superconducting, layer in the vicinity of the topological surface state, which could serve to incorporate some of the novel properties of topological insulators into device applications. Furthermore, apart from its interaction with the topological state, the 2DEG, existing in a material characterised by a very large spin-orbit interaction, could itself find application in spintronic devices [40] . However, the increase in scattering rate of the topological state that we observe following creation of the 2DEG also suggests that the additional decay channels that this opens up could be detrimental to some applications of topological insulators. The conducting surface-localized 2DEG will also have a large influence on transport measurements. We stress that the new states which we report here are not additional surface states of the form observed in Bi 1− x Sb x alloys [4] . Rather, they reflect the electronic structure of the quantum-confined electron gas residing in the quantum well defined by the surface band bending and the vacuum. As both scenarios give rise to electronic states with no dispersion along the surface normal, care must be taken to distinguish between 2DEG and conventional surface states in ARPES measurements. Here, the appearance of the states concurrent with a downward shift of the Dirac point, the similarity of their in-plane dispersion to that of the bulk conduction band, the particular resonance behaviour of the photoemission that we observe from these states, and the model calculations together unambiguously classify them as 2DEG states associated with a downward surface band bending. Equivalent resulting band bending effects as those observed here could be expected across a wide range of similar materials, suggesting 2DEGs represent a hitherto unreported additional characteristic surface effect of topological insulators. Sample growth Single crystals of Bi 2 Se 3 were grown as follows: Stoichiometric mixtures of 5N purity elemental Bi and Se were melted at 860 °C for 24 h in an evacuated quartz ampoule, cooled down to 650 °C at a rate of 2.5 °C h−1, and then annealed at 650 °C for another two days. The sample was then removed to another evacuated quartz ampoule with a conical bottom and zone melted through an induction coil with a rate of 1.2 mm h−1. Angle-resolved photoemission measurements Angle-resolved photoemission measurements were performed at the SGM-3 beamline of the ASTRID synchrotron radiation facility in Aarhus. The samples were cleaved at room temperature and ARPES data were taken at around 60 K. Between cleaving and the reported measurements, the sample temperature was thus above 60 K, such that the more rapid change in the Fermi energy compared to that reported by Hsieh et al . [13] can be explained by the higher sample temperature. For the detailed mapping of the states, the energy and angular resolutions were set to better than 10 meV and 0.13°, respectively. The photon energy for the data in Figures 1 and 3 was 16 eV. For the photon energy scan in Figure 2 , the energy resolution was better than 20 meV. The k z values for the three-dimensional representation of the photon energy scan of Figure 2 were calculated using free-electron final states, i.e., , where Θ is the emission angle and V 0 is the inner potential, chosen to be 11.8 eV, in good agreement with ref. 14 . The intensity of each individual image has been normalized such that the maximum amount of detail is visible in the k z maps. 2DEG calculations The coupled Poisson-Schrödinger calculations [38] were performed incorporating both the non-parabolicity of the conduction band dispersion as well as the anisotropy of the effective mass along different crystallographic directions. The in-plane mass was taken as 0.122 m 0 and 0.109 m 0 along the directions, respectively, where m 0 is the free-electron mass. Along k z , an effective mass of 0.24 m 0 was used, estimated from the bulk conduction band dispersion shown in Figure 2a . The band gap was taken as 350 meV, and a bulk dielectric constant of 113 was used. The bulk carrier density was set at 2.45×10 19 cm −3 , corresponding to a bulk Fermi level 0.16 eV above the conduction band edge, as estimated from the ARPES data. How to cite this article: Bianchi, M. et al . Coexistence of the topological state and a two-dimensional electron gas on the surface of Bi 2 Se 3 . Nat. Commun. 1:128 doi: 10.1038/ncomms1131 (2010).